Genome-wide association study reveals two new risk loci for bipolar disorder Bipolar disorder (BD) is a common and highly heritable mental illness and genome-wide association studies (GWAS) have robustly identified the first common genetic variants involved in disease aetiology. The data also provide strong evidence for the presence of multiple additional risk loci, each contributing a relatively small effect to BD susceptibility. Large samples are necessary to detect these risk loci. Here we present results from the largest BD GWAS to date by investigating 2.3 million single-nucleotide polymorphisms (SNPs) in a sample of 24,025 patients and controls. We detect 56 genome-wide significant SNPs in five chromosomal regions including previously reported risk loci ANK3 , ODZ4 and TRANK1, as well as the risk locus ADCY2 (5p15.31) and a region between MIR2113 and POU3F2 (6q16.1). ADCY2 is a key enzyme in cAMP signalling and our finding provides new insights into the biological mechanisms involved in the development of BD. Bipolar disorder (BD) is a severe disorder of mood, characterized by recurrent episodes of mania and depression, which affect thought, perception, emotion and social behaviour. With a lifetime prevalence of 1% in the general population, BD is a common condition. The World Health Organisation classifies BD as one of the top 10 leading causes of the global burden of disease for the age group of 15–44-year-old people. Formal and molecular genetic data strongly suggest that BD is a multifactorial disease [1] . This means that many genetic and environmental factors influence the risk of disease. The heritability estimates for BD range between 60 and 80% [2] . This suggests a substantial involvement of genetic factors in the development of the disease, but the particular factors underlying the pathophysiology and aetiology of BD are still largely unknown. Since the first genome-wide association study (GWAS) of BD [3] in 2007, a handful of risk loci have been identified through some larger GWAS, which replicated in adequately sized follow-up studies [4] , [5] , notably ANK3 , NCAN , CACNA1C and ODZ4. These first genes provide valuable insights into the molecular mechanisms involved in BD and form a basis for future exploration of the molecular pathomechanisms and possibly drug targets. The genetic risk variants at these loci show unprecedented statistical support, but explain only a smaller fraction of BD’s heritability. However, this is in line with results of recent studies that provide evidence for a strong polygenic component in BD, suggesting the presence of a large number of additional risk loci, each mediating small disease susceptibility [6] , [7] . Motivated by this and the successes of GWAS for non-psychiatric phenotypes, a big step forward was taken through a recent large BD GWAS by the multi-national Psychiatric Genomics Consortium Bipolar Disorder Working Group (PGC-BD) [7] . We have previously published a GWAS of BD using a German sample (named Germany I) [8] that was thereafter included in the GWAS of the PGC-BD [7] and another subsequent BD GWAS [9] . Here we generate new and so far unpublished genome-wide SNP data from 2,266 clinically well-characterized patients with BD ( ∼ 76% BD type I) and 5,028 ethnically matched controls, derived from the MooDS (Systematic Investigation of the Molecular Causes of Major Mood Disorders and Schizophrenia) consortium. The samples originate from four European countries, Canada and Australia. To increase power for detection of risk variants with small genetic effect, we combine and jointly analyse our MooDS samples with the 7,481 patients and 9,250 controls from the aforementioned PGC-BD study (MooDS-PGC). We find strong evidence for common risk variants at three known loci ( ANK3 , ODZ4 and TRANK1 ) and identify two risk loci ( ADCY2 and the region between MIR2113 and POU3F2 ), which have not been implicated in BD before. 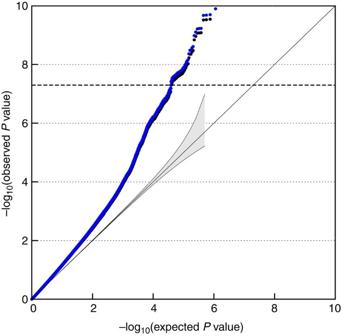Figure 1: Quantile–quantile plot of the MooDS-PGC GWAS of BD. A quantile–quantile (QQ) plot displays the relationship between the experimentally observedPvalues (vertical axis) to the expectedPvalues of a null distribution (horizontal axis). The grey area represents the 95% concentration band. QQ plots are commonly used for graphical illustration of the effect of a QC on GWAS data. The dashed line (bold) indicates the threshold for genome-wide significance (PGC=5 × 10−8). Here we show the effect of a standardisedλfactor for GC on the 2,267,487 autosomalPvalues from the fixed-effects meta-analysis (blue curve) in the last step of our QC procedure (Methods). After the application, a systematic adjustment ofPvalues (PGC, black curve) can be seen, suggesting that this QC step counteracts an inflation ofPvalues by varying sample sizes in the MooDS and PGC data. Association analyses A total of 2,267,487 imputed SNPs from 9,747 patients and 14,278 controls ( Table 1 ) passed our stringent quality control (QC) and association analysis of autosomal SNPs was performed using a fixed-effects meta-analysis (Methods). Sex chromosomes were not analysed because the published PGC data do not contain the respective information. To adequately correct for inflation of P values due to varying sizes of the MooDS and PGC samples, we adjusted the P values of the MooDS-PGC analysis ( P GC ) using a standardized λ factor for genomic control (GC), which was 1.018 (Methods, Fig. 1 ). A P value plot showing an overview of the genome-wide association results is provided in Fig. 2a . Table 1 Phenotypic data for patients with bipolar disorder and controls following QC. Full size table Figure 1: Quantile–quantile plot of the MooDS-PGC GWAS of BD. A quantile–quantile (QQ) plot displays the relationship between the experimentally observed P values (vertical axis) to the expected P values of a null distribution (horizontal axis). The grey area represents the 95% concentration band. QQ plots are commonly used for graphical illustration of the effect of a QC on GWAS data. The dashed line (bold) indicates the threshold for genome-wide significance ( P GC =5 × 10 −8 ). Here we show the effect of a standardised λ factor for GC on the 2,267,487 autosomal P values from the fixed-effects meta-analysis (blue curve) in the last step of our QC procedure (Methods). After the application, a systematic adjustment of P values ( P GC , black curve) can be seen, suggesting that this QC step counteracts an inflation of P values by varying sample sizes in the MooDS and PGC data. 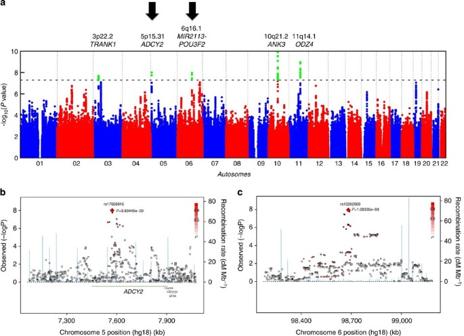Figure 2: Association results for the MooDS-PGC GWAS and the two new risk loci for BD. (a) Manhattan plot for all analysed SNPs, (b,c) regional association plots for the SNPs analysed atADCY2(5p15.31) andMIR2113-POU3F2(6q16.1). Regional association plots were drawn using SNAP54and data for LD (red) and recombination frequency (blue line) from the 1000 Genomes Project. Full size image Figure 2: Association results for the MooDS-PGC GWAS and the two new risk loci for BD. ( a ) Manhattan plot for all analysed SNPs, ( b , c ) regional association plots for the SNPs analysed at ADCY2 (5p15.31) and MIR2113 - POU3F2 (6q16.1). Regional association plots were drawn using SNAP [54] and data for LD (red) and recombination frequency (blue line) from the 1000 Genomes Project. Full size image The MooDS-PGC GWAS revealed 56 SNPs reaching genome-wide significance at five genomic loci, three of which had been described before ( ANK3 , ODZ4 and TRANK1 ) [4] , [9] . A subset of 18 non-correlated top SNPs, which were selected by a pruning on pairwise linkage disequilibrium (LD) between the associated SNPs, is provided in Table 2 . Full lists of SNPs with evidence of strong-to-moderate association ( P GC <5 × 10 −5 ) are given in Supplementary Tables 1–5 . Table 2 Eighteen GWAS SNPs showing genome-wide evidence for association with BD in the combined MooDS and PGC samples. Full size table Overall, the most significant association signal and the largest number of genome-wide significant SNPs ( n =26) were identified in ANK3 (ankyrin 3) on chromosome 10q21.2 (top: rs10994415-C, P GC =6.88 × 10 −11 , OR=1.27). SNP rs10994415 is in moderate LD with rs10994397 ( r 2 =0.62), which is the most significant finding for ANK3 in the original PGC-BD study [7] and the second most significant finding in this GWAS ( P GC =2.86 × 10 −10 , OR=1.29). Additionally, rs10994415 is in strong LD with rs1938526 ( r 2 =0.79) and in moderate LD with rs10994336 ( r 2 =0.47), both genome-wide significant ( P GC =8.55 × 10 −10 , OR=1.27; P GC =2.34 × 10 −8 , OR=1.27) and originally found as BD risk variants by Ferreira et al. [10] Our second most significant locus was marked by 10 genome-wide significant SNPs in ODZ4 (odd Oz/ten-m homologue 4 alias teneurin transmembrane protein 4, TENM4 ) on chromosome 11q14.1 (top: rs12290811-A, P GC =1.09 × 10 −09 , OR=1.19). rs12290811 was first described by Ferreira et al. [10] with suggestive evidence for association with BD [10] . This SNP is in moderate LD with ODZ4 rs12576775 ( r 2 =0.57, P GC =4.46 × 10 −9 , OR=1.17), the second best finding of the PGC-BD study [7] with genome-wide significance (after their CACNA1C rs4765913 finding). As the third and fourth most significant finding in our study, we discovered two previously undescribed risk loci for BD. On chromosome 5p15.31, two genome-wide significant SNPs are located in ADCY2 (adenylate cyclase 2, top: rs17826816-G, P GC =9.89 × 10 −9 , OR=1.14) and four were found in a region between the genes MIR2113 (microRNA 2113) and POU3F2 (POU class 3 homeobox 2) on chromosome 6q16.1 (top: rs12202969-A, P GC =1.08 × 10 −8 , OR=1.12). P value plots that provide a regional overview of the associated SNPs as well as OR plots that show the effect sizes of the top variant in each subsample are provided in Figs 2b, and 3a,b . A comprehensive lookup of previous findings at these loci in the catalogue of published GWAS [11] (as of 4 October 2013) and literature a search did not provide any genome-wide significant GWAS finding for BD in windows of 1 Mb around the top SNPs. 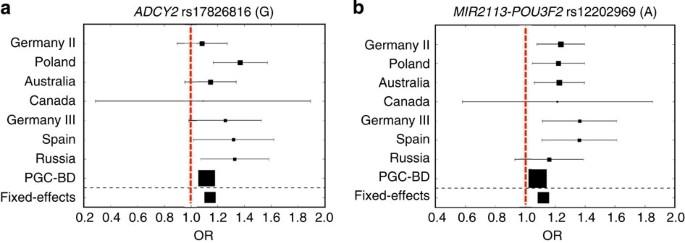Figure 3: Genetic effect sizes for the two new risk loci identified through the MooDS-PGC GWAS of BD. (a,b) Forest plots displaying the most significant SNP’s odds ratio (OR, full square) and their 95% confidence interval (horizontal continuous lines) for the geneADCY2(5p15.31) as well as the region between the genesMIR2113andPOU3F2(6q16.1). The overall OR was calculated using a fixed-effects meta-analysis based on the weightedz-score method51. The effect allele of each SNP is given in brackets. The area of a square reflects the statistical power of the respective study sample. Areas were calculated by the reciprocal value of the standard deviations. Figure 3: Genetic effect sizes for the two new risk loci identified through the MooDS-PGC GWAS of BD. ( a , b ) Forest plots displaying the most significant SNP’s odds ratio (OR, full square) and their 95% confidence interval (horizontal continuous lines) for the gene ADCY2 (5p15.31) as well as the region between the genes MIR2113 and POU3F2 (6q16.1). The overall OR was calculated using a fixed-effects meta-analysis based on the weighted z -score method [51] . The effect allele of each SNP is given in brackets. The area of a square reflects the statistical power of the respective study sample. Areas were calculated by the reciprocal value of the standard deviations. Full size image Another known BD risk locus with genome-wide significance was TRANK1 (tetratricopeptide repeat and ankyrin repeat containing 1 alias lupus Brain antigen 1 homologue, LBA1 ) on chromosome 3p22.2, which was the fifth best-supported locus in our study (top: rs6550435-G, P GC =2.05 × 10 −8 , OR=1.13). rs9834970, a SNP in low LD ( r 2 =0.13, P GC =4.81 × 10 −8 , OR=1.12), had already reached genome-wide significance in a GWAS of BD by Chen et al. [9] , which partially overlaps with the included PGC data. Analysis of rs9834970-C in MooDS showed P GC =0.0014 (OR=1.15), providing independent evidence for replication. NCAN (neurocan) on chromosome 19p13.11 was identified as a genome-wide significant risk locus for BD in the first MooDS study [8] . In our present analysis, a SNP in strong LD with the original SNP rs1064395 ( r 2 =0.96) showed a sub-genome-wide significant result (rs2011503-C, P GC =8.79 × 10 −8 ; OR=0.87). CACNA1C (calcium channel, voltage-dependent, L type, alpha 1C subunit) on chromosome 12p13.33 was originally described as BD risk locus in the study by Ferreira et al. [10] ; in fact, SNPs rs1006737 and rs1024582 were found at the border of genome-wide significance. CACNA1C received additional support in the PGC-BD study [7] and a subsequent study by Green et al. [12] , in which rs4765913, a SNP with moderate LD to rs1006737 and rs1024582 ( r 2 =0.40 and r 2 =0.49), was genome-wide significant. In the present MooDS-PGC analysis, rs4765913 was the most significant CACNA1C finding but failed to reach genome-wide significance (rs4765913-A, P GC =9.69 × 10 −6 , OR=1.12). None of these three known CACNA1C risk variants was supported by the new MooDS data (rs4765913-A, P MooDS =0.568, OR=1.03; rs1006737-A, P MooDS =0.643, OR=1.02; rs1024582-A; P MooDS =0.614, OR=1.02). Regional association plots for the known risk loci ( ANK3 , ODZ4 , TRANK1 , NCAN and CACNA1C ) are provided in Supplementary Fig. 1a–e . Follow-up analyses To characterize our new findings in silico , we have looked up relevant databases for prior knowledge about the SNPs and genes. At both loci, we screened all SNPs with strong-to-moderate evidence for association ( P GC <5 × 10 −5 , Supplementary Tables 3 and 4 ) for potentially functional effects such as missense variants with a consequence on the protein’s primary structure or variants with an effect on expression in different body tissues including important brain regions. To broaden the search range in data from prior studies or databases that did not contain the original SNP from our analysis, we have also included proxy SNPs that are in strong LD with the analysed GWAS SNPs ( r 2 >0.8, Supplementary Tables 6 and 7 ). For the 5p15.31 locus, the top SNP rs17826816 is located in intron 2 of the largest protein-coding transcript of ADCY2 (RefSeq NM_020546.2, Ensembl ENSG00000078295). This transcript (Ensembl ENST00000338316) has a length of 6,575 base pairs and contains 25 exons that encode 1,091 amino-acid residues (UniProt Q08462, Ensembl ENSP00000342952). rs13166360 ( P GC =1.81 × 10 −8 ; OR=1.14), a proxy for rs17826816 ( r 2 =0.95) and the other genome-wide significant SNP in the gene, is located in exon 3 where it mediates an amino-acid change of the nonpolar residue valine to the hydrophobic residue leucine at position 147. rs13166360 impacts on the fourth α-helix of the first transmembrane domain. This missense variant has been predicted as possibly damaging for the protein by a HumDiv data-trained PolyPhen-2 (ref. 13 ) analysis. For the 6q16.1 locus, the associated variants that are located closest to the neighbouring genes are rs9385269 (P GC =8.74 × 10 −7 , OR=1.10) with a distance of 75 kb to MIR2113 and rs9375371 (P GC =5.33 × 10 −6 , OR=1.11) with a distance of 531 kb to POU3F2 . We did not find a variant in strong LD ( r 2 >0.8) that is directly located in either of the two genes. The genome-wide significant top SNP (rs12202969) is located 104 kb downstream of MIR2113 and 706 kb upstream of POU3F2 . To further explore the region between both genes, we investigated ENCODE [14] data at the UCSC Genome Browser [15] as well as data from GTEx [16] , PheGenI [17] , RegulomeDB [18] , seeQTL [19] and an expressed quantitative trait locus (eQTL) browser by the Pritchard lab ( http://eqtl.uchicago.edu/cgi-bin/gbrowse/eqtl/ ). We did not find robust evidence for an eQTL. However, in RegulomeDB, we found suggestive evidence that rs10457441 ( P GC =4.99E-07, OR=1.11) overlaps with regulatory DNA features such as open chromatin, histone modifications and binding sites for the transcription factors (EP300, USF1 and STAT3). Besides that, rs1906252 ( P GC =3.39 × 10 −8 ; OR=1.12), which is in strong LD with the top SNP (rs12202969), was among the most significant finding in a GWAS of information processing speed (measured by a symbol search test in 991 healthy elderly probands from Scotland) [20] . Since an enrichment of association signals in target genes for MIR137 has been observed in schizophrenia [4] , we also tested whether known or predicted targets of MIR2113 are enriched for significant P values, but did not find support for this hypothesis. The present GWAS is based on 24,025 patients and controls and combines so far unpublished MooDS samples with the published PGC-BD GWAS samples. Our study adds two new risk loci, namely the gene ADCY2 and the 6q16.1 region, to the list of known BD risk loci identified through GWAS ( ANK3 , NCAN , CACNA1C and ODZ4 ). The MooDS data provide strong statistical support for three of these loci, except for CACNA1C . Several lines of evidence support an involvement of the two new loci in the neurobiology of BD and major psychiatric disorders. For some variants, functional effects on DNA and protein levels are suggested using knowledge from bioinformatical resources. Our finding in the 6q16.1 region is located within a linkage peak identified by independent genome scans in BD families [21] . The genome-wide significant top SNP from our GWAS (rs12202969) is located downstream of an uncharacterized microRNA gene ( MIR2113 ) and upstream of a transcription factor gene ( POU3F2 ) that has been found to contribute to neocortex development in mice [22] . Using all available proxies for the SNPs with highly to moderately significant evidence for association, we did not find a variant in a gene in LD. However, one of the four genome-wide significant SNPs in the region (rs1906252) was found to be associated with a cognitive phenotype, speed of information processing, in an independent GWAS [20] . In addition, one SNP below genome-wide significance (rs10457441) converges with DNA features that are indicative for a potential involvement in gene expression regulation. The ADCY2 gene on chromosome 5p15.31 is expressed in the brain and encodes a cell membrane-bound enzyme for the synthesis of the second-messenger molecule cAMP. The ADCY2 protein is primarily regulated by heterotrimeric G proteins and produces cAMP in response to extracellular hormones and neurotransmitters that bind as ligands to G protein-coupled receptors (GPCRs) [23] . ADCY2 is also regulated by the protein kinase C (PKC) and the RAF kinase. ADCY2 is insensitive to calcium ions and calmodulin; both are regulators of other adenylate cyclases. cAMP induces the expression of downstream target genes by activation of the cAMP-dependent protein kinase A (PKA) and subsequent phosphorylation of the transcription factor cAMP response element-binding protein (CREB) [24] . GPCRs represent the majority of neurotransmitter receptors for dopamine, norepinephrine and serotonin, and belong to the earliest functional candidate genes for neuropsychiatric disorders. One of our two genome-wide significant SNPs in ADCY2 is a missense variant with possibly damaging effect on the protein (rs13166360). We speculate that functional variation in ADCY2 may have a more pronounced effect on BD susceptibility than functional variation in neurotransmitter receptors where a high degree of redundancy may facilitate functional compensation of one dysfunctional receptor by another. In a recent co-expression network analysis for the human brain transcriptome, ADCY2 showed up among the top 50 of 310 genes, which altogether form a network module specific for postnatal telencephalon (neocortex, hippocampus, amygdala and striatum) [25] . Those top (or ‘hub’) genes show the highest network connectivity within the module and should therefore have the highest potential functional relevance for these brain regions. For SNPs located in 2 of the top 10 hub genes, independent GWAS have found strong association with schizophrenia (neurogranin, NRGN ) [26] and increasing suicidality in major depression (guanine deaminase, GDA ) [27] , two psychiatric disorders that partially share genetic risk factors with BD [28] . Data from the Stanley Medical Research Institute Online Genomics Database [29] show a 1.5–2.0-fold lower ADCY2 expression in Brodmann areas 10 and 46 (BA10/46) of patients with BD as well as in patients with major depression disorder compared with controls ( P <0.01). Noteworthy, data from the same resource indicate that expression levels of CACNA1C , ODZ4 and NCAN in these two areas are also significantly reduced in patients with BD and depression. BA10/46 map to neighbouring frontal and middle frontal regions in the prefrontal cortex and abnormalities in these brain areas have been described in both disorders [30] , [31] . In summary, our study implicates common variation at two genomic loci as new genetic risk factors for BD. While a specific gene cannot be pinned down at one of the risk loci (6q16.1), it harbours a genome-wide significant SNP that was previously shown to be associated with variation of the ‘information processing speed’, a cognitive function that has been postulated as a valid and highly specific cognitive endophenotype for BD, differentiating both euthymic BD patients and their healthy first-degree relatives from healthy controls [32] . ADCY2 plays a key role in cAMP-dependent GPCR pathways. Disturbed neurotransmission at these pathways is a long-standing hypothesis in psychiatric research, which has motivated multiple candidate gene studies. Most of these studies, however, focused on variation in neurotransmitter receptor and transporter genes and less on adenylate cyclase genes, located more downstream and bundling the signals coming in from several neurotransmitter receptor types. Adenylate cyclase may therefore represent a functional bottleneck in signal transduction pathways and genetic variation may have a more direct influence on the phenotype than at positions with higher functional redundancy (neurotransmitter receptors/transporters). This may also explain the somewhat surprising observation that GWAS in neuropsychiatric disorders performed so far did not identify strong association signals in neurotransmitter/transporter genes. Phenotypic data of the study samples Written informed consent was obtained from all patients and controls before participation in the study. Protocols and procedures were approved by the local Ethics Committees of the hospitals mentioned below. An overview of the phenotyping of the seven new MooDS samples and the PGC-BD GWAS sample are provided in Table 1 . For MooDS patients, affected subjects received a lifetime diagnosis of BD (type I, type II, schizoaffective disorder bipolar type, BD not otherwise specified) according to DSM-IV [33] criteria using a consensus best-estimate procedure [34] and structured interviews [35] , [36] . Patients were recruited from consecutive admissions to psychiatric in-patient units at the University Hospital Würzburg (Germany II), at the Central Institute of Mental Health in Mannheim and other collaborating psychiatric hospitals in Germany (Germany III), at the Mood Disorder Unit, Prince of Wales Hospital in Sydney (Australia), at the Department of Psychiatry, Poznan University of Medical Sciences (Poland), at specialty mood disorders clinics in Halifax and Ottawa (Canada), at the Russian State Medical University, Moscow (Russia), and at the Civil Hospital Carlos Haya, Málaga (Spain). For MooDS controls, unaffected subjects were drawn from the population-based Heinz Nixdorf Recall (HNR) Study [37] (Germany II), from a Munich-based community sample by the Max Planck Institute of Psychiatry [38] (Germany III), from parents of adolescent twins by the Brisbane Longitudinal Twin Study and a community sample (Australia), from a hospital-based sample by the University of Szczecin (Poland), from a combined sample by the Saguenay-Lac-Saint-Jean (SLSJ) study (Canada), from a combined sample by the Kursk State Medical University (KSMU) study and the UFA study (Russia), and from parts of the European Community Respiratory Health Survey (ECRHS) (Spain). Controls for the Russian sample were generated by GABRIEL, a multidisciplinary study to identify the genetic and environmental causes of asthma in the European Community [39] . The Canadian and Spanish controls were kindly provided by Catherine Laprise (UQAC, Saguenay, Canada) and Manolis Kogevinas (CREAL, Barcelona, Spain). Polish controls were produced by the International Agency for Research on Cancer (IARC) and the Centre National de Génotypage (CNG) GWAS Initiative for a study of upper aerodigestive tract cancers [40] . Except the controls for Germany III, none of the above-mentioned controls were screened for the presence of a neuropsychiatric phenotype. Genetic data of the study samples Over the last 5 years, the MooDS consortium produced two waves of genome-wide data for BD. The first wave of data (Germany I) were generated for the GWAS by Cichon et al. [8] and are now part of the PGC-BD GWAS data [7] . The second wave of data were generated for the present GWAS and are described below. For Polish, Canadian, Russian and Spanish patients, lymphocyte DNA was isolated from EDTA anti-coagulated venous blood by salting-out with saturated sodium chloride solution [41] or by a Chemagic Magnetic Separation Module I (Chemagen, Baesweiler, Germany) according to the manufacturer’s recommendations. DNA samples were genome-wide genotyped using Infinium assays (Illumina, San Diego, CA, USA) for BeadChips Human660W-Quad (Polish patients) and HumanOmni1-Quad (Canadian, Russian and Spanish patients). DNA extraction and genotyping was performed at the Department of Genomics, Life & Brain Center, University of Bonn, Germany. Genome-wide genotyped data for Russian and Polish controls were available from previous studies of asthma and cancer [39] , [40] . Canadian and Spanish data were kindly provided by Catherine Laprise (UQAC, Saguenay, Canada) and Manolis Kogevinas (CREAL, Barcelona, Spain). Genotyping of the samples Australia, Germany II, Germany III, and PGC-BD were described in previous studies [7] , [8] , [42] , [43] , [44] . We aimed to genotype the patient and controls from the same population on the same chip type. However, depending on the chip type that was commercially available at the time of our genotyping, respectively, which has been used by other studies from which we have drawn data, some samples were genotyped on different BeadChips. For the seven new MooDS samples, the predominant chip types were the Human610-Quad and the HumanOmni1-Quad. The other chip types were the HumanHap550, the Human660Q-Quad and the HumanHap300. Supplementary Table 8 summarizes the genotyping chips for all new MooDS samples. In the PGC study [7] , SNP genotypes from 11 individual GWAS samples were imputed up to a set of more than two million autosomal markers using reference haplotypes from the HapMap phase 2 CEU sample. To produce a fitting marker set for the seven MooDS samples, the SNPs of each MooDS sample were pruned to the least common set (first and second QC) before the imputation (see below) and subsequent sample-specific association analyses (followed by a third QC). After the alignment of the MooDS and the PGC sets and another filtering step, the final SNP sets were carried on to the meta-analysis. The first and second QC was performed using several tools from INTERSNP [45] (version 1.11) and PLINK [46] (version 1.07) as described below. The third QC consisted of manual filtering of data from IMPUTE [47] (version 2) and SNPTEST [48] (version 1). Supplementary Data 1 illustrate the steps of the QC procedure and the numbers of subjects and SNPs excluded at each individual step. In particular, the first QC comprised five filtering steps (exclusion criteria are given in brackets) and was performed for each sample separately. We investigated SNP and subject call rates (CR<95% and CR<98%), sex status of each subject (inconsistency between data from recruitment centres and X-chromosome heterozygosity rate), deviation of a SNP from the Hardy–Weinberg Equilibrium ( P ≤1 × 10 −6 ) and cryptic relatedness between pairs of subjects (identity-by-state (IBS) >1.98 or s.d. six times higher than the IBS averaged over all pairs of the sample). If patients and controls have been genotyped on different chip types, the SNP set was reduced to those SNPs available in patients and controls after the first QC. In this way, we avoided potential differential error that have could arised from SNPs that are genotyped in patients but imputed in controls, or vice versa . The second QC consisted of another five filtering steps, that is, SNPs with coding conflicts between SNP sets of different chip types (A/T and G/C SNPs), potential population stratification within and between samples using multi-dimensional scaling analysis (MDS, identification of population outliers by visual assessment, Supplementary Fig. 2 ), subjects with an excess of heterozygosity (inbreeding coefficient >4 s.d. from the sample’s mean), cryptic relatedness (IBS>1.98 or s.d.>6) and monomorphic SNPs (MAF<0.01%). We assessed the effect of the first and second QC on the genotype data by a calculation of a genomic inflation factor λ . Each sample showed λ ≤1.05. Imputation of the MooDS data sets was carried out using IMPUTE and the February 2012 release of the 1,000 Genomes Project data [49] . Imputed SNPs with an info score <0.4 or a MAF <0.03 were removed during the third QC and the sample-specific association analyses (see below). We aligned the imputed SNP sets between MooDS and PGC and excluded SNPs that were absent in three or more MooDS samples and/or were not present in the PGC, resulting in a number of 2,267,487 autosomal SNPs for 2,266 patients and 5,028 controls from MooDS, and 9,747 patients and 9,250 controls from PGC. Finally, we assessed the effect of the QC procedure by further calculations of genomic inflation factors. The λ values for a standardized sample size of 1,000 patients and 1,000 controls and the non-standardized λ values were 1.027 and 1.084 for MooDS, 1.018 and 1.147 for PGC, and 1.018 and 1.203 for the combination of both. As ancestry was assigned to patients and controls on the basis of self-reported ancestry, we inspected the ethnical matching between patients and controls within and between the MooDS samples by a MDS analysis. After exclusion of population outliers (described above), we used the significant MDS dimensions used as covariates in the sample-specific association analyses that were conducted using SNPTEST. Using the eight quality-controlled samples for MooDS and PGC, meta-analysis was performed with YAMAS [50] under a fixed-effects model. For each SNP, effect estimates and their s.e. were combined across the eight data sets as described elsewhere [51] . To adequately correct for inflation of P values due to varying sample sizes, we adjusted the P values for the MooDS-PGC analysis ( P GC ) using the standardized λ factor for GC, which was 1.018 (described above). We considered an association as genome-wide significant if P GC <5 × 10 −8 . Overlap between new samples and previous BD studies It is noteworthy that none of the seven MooDS samples have been analysed in a genome-wide discovery step for BD before. However, parts of Poland, Spain and Russia have been used for targeted genotyping of 48 SNPs for the first replication step of our previous GWAS of BD [8] . Parts of Australia and Germany III have been used for the second replication step of that study [8] , that is, extraction of one SNP from genome-wide data. Thirty eight SNPs from the genome-wide data of Germany II, Germany III (alias BOMA-Rep1 and BOMA–Rep2) and Australia have been used in the replication step of the previous PGC study [7] . The Canadian patients partially overlap with a linkage and expression study of BD [52] and a candidate gene association study of BD [53] . How to cite this article: Mühleisen, T. W. et al. Genome-wide association study reveals two new risk loci for bipolar disorder. Nat. Commun. 5:3339 doi: 10.1038/ncomms4339 (2014).